High transconductance organic electrochemical transistors The development of transistors with high gain is essential for applications ranging from switching elements and drivers to transducers for chemical and biological sensing. Organic transistors have become well-established based on their distinct advantages, including ease of fabrication, synthetic freedom for chemical functionalization, and the ability to take on unique form factors. These devices, however, are largely viewed as belonging to the low-end of the performance spectrum. Here we present organic electrochemical transistors with a transconductance in the mS range, outperforming transistors from both traditional and emerging semiconductors. The transconductance of these devices remains fairly constant from DC up to a frequency of the order of 1 kHz, a value determined by the process of ion transport between the electrolyte and the channel. These devices, which continue to work even after being crumpled, are predicted to be highly relevant as transducers in biosensing applications. High gain is a requirement for transistors in a broad range of applications. In sensors, for example, high gain is associated with high sensitivity, as a small signal in the transistor input yields a large response in the output. There is a tremendous effort to make these devices from soft materials, where low-cost or high-throughput fabrication is desired or where mechanical compatibility with soft tissue is required. The advantageous properties of organic electronic materials, including versatility in processing and synthetic tunability, have allowed for a variety of applications where organic electronic devices are poised to disruptively overtake existing technologies [1] . A particular organic transistor configuration that is currently attracting a great deal of attention is the organic electrochemical transistor (OECT). Originally developed by White et al . [2] , OECTs use an electrolyte as an integral part of their device structure. These devices hold considerable promise for technologies such as medical diagnostics and bioelectronic implants due to improved biological and mechanical compatibility with tissue compared with traditional ‘hard’ electronic materials [3] , [4] . OECTs have recently been employed in chemical and biological sensing [5] , and have also been interfaced with cells to control cell adhesion [6] , and to monitor cell viability [7] and barrier tissue integrity [8] . OECTs have been fabricated using low-cost printing techniques [9] , and integrated with natural [10] and synthetic fibres [11] in powerful demonstrations of the unique form factors that can be achieved with these devices. In addition, OECTs utilizing solid or gel electrolytes have widened the scope of application [12] , showing promise as printable logic circuits [13] , and drivers for haptic sensors [14] and flat panel display pixels [15] . In most of these applications, transistors convert a modulation in the gate voltage Δ V G to a modulation in the drain current Δ I D . The figure-of-merit that determines this conversion is the transconductance, defined as g m =Δ I D /Δ V G . The transconductance is the main transistor parameter that governs signal amplification: a simple voltage amplifier, for example, can be built by connecting a resistor R in series with the drain. The voltage amplification (voltage modulation across the resistor versus voltage modulation at the gate) is equal to g m R . Despite their many attractive characteristics, transistors based on organic semiconductors are generally not known for their high transconductance, but are instead dismissed in favour of traditional inorganic semiconductors, and, more recently, oxide and graphene-based devices. In this work, we present mechanically flexible OECTs with a transconductance that exceeds that of all other electrolyte-gated transistors and most solid-state devices made of inorganic and low-dimensional nanowire and carbon-based semiconductors. Structure of the transistors The device architecture of the OECTs developed for this work is shown in Fig. 1 . The channel consists of a 400-nm thick film of the conducting polymer poly(3,4-ethylenedioxythiophene) doped with poly(styrene sulphonate) (PEDOT:PSS), deposited from a commercially available aqueous dispersion and patterned using photolithography. In this material, PEDOT is a semiconductor, which is degenerately doped p- type by PSS to reach conductivities as high as 1,000 S cm −1 . Gold source and drain contacts, also patterned photolithographically, define the channel length. The channel length, L , is varied between 5 and 10 μm, and the width, W , is 10 μm. A 2-μm-thick parylene-C film insulates the contacts from the electrolyte solution, and defines an opening where the channel is in direct contact with the electrolyte (a 100-mM NaCl solution). A Ag/AgCl wire immersed in the electrolyte is used as the gate electrode. 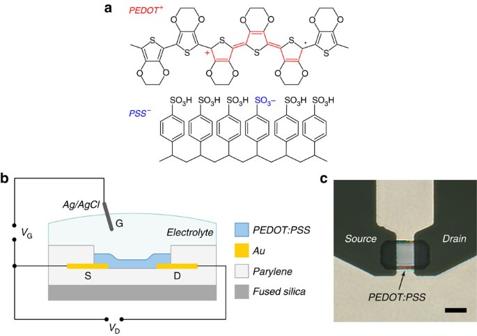Figure 1: Active material and structure of the transistor. (a) Chemical structure of PEDOT and PSS. A hole, indicated as a positive polaron on the PEDOT chain, is compensated by a sulphonate ion on the PSS chain. (b) Schematic of an OECT cross-section and the wiring diagram for device operation. (c) Optical micrograph of an individual transistor. Scale bar, 10 μm. Figure 1: Active material and structure of the transistor. ( a ) Chemical structure of PEDOT and PSS. A hole, indicated as a positive polaron on the PEDOT chain, is compensated by a sulphonate ion on the PSS chain. ( b ) Schematic of an OECT cross-section and the wiring diagram for device operation. ( c ) Optical micrograph of an individual transistor. Scale bar, 10 μm. 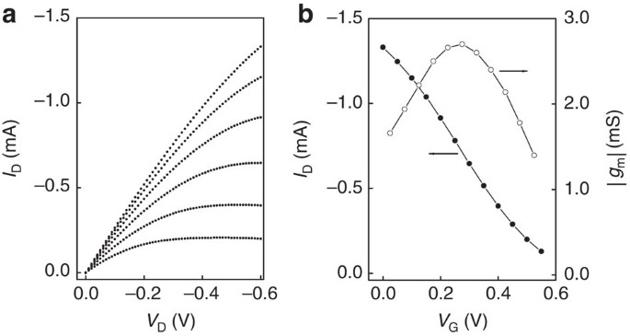Figure 2: Steady-state characteristics. (a) Output characteristics forVGvarying from 0 (top curve) to +0.5 V (bottom curve) with a step of +0.1 V. (b) Transfer curve forVD=−0.6 V, and the associated transconductance. Full size image Steady-state characteristics Figure 2 shows the output characteristics of a typical OECT ( L =5 μm, W =10 μm) with negative bias at the drain, V D , and for gate bias, V G , varying from 0 to +0.5 V. These characteristics show the low voltage operation that is the hallmark of electrolyte-gated transistors. The time delay between sourcing V D and V G and measuring the drain current ( I D ) was 100 ms, which was found to be significantly longer than the time required for the drain current to reach steady-state. The gate current, also measured after the same delay, was <10 nA for V D =−0.6 V and V G =+0.5 V. The corresponding transfer curve for V D =−0.6 V is shown in Fig. 2 . The drain current decreases with gate voltage, consistent with operation in the depletion regime. This behaviour is in agreement with our current understanding of the operation mechanism of OECTs [16] : when a positive bias is applied at the gate, cations from the electrolyte enter the PEDOT:PSS film and compensate the pendant sulphonate anions on the PSS. This leads to a decrease of the hole density in the PEDOT, as holes extracted at the drain are not re-injected at the source. The end result is the decrease of the drain current seen in Fig. 2 . This effect is analogous to compensation doping of a p- type semiconductor upon the implantation of donors, but occurs in OECTs at room temperature and at a low applied bias. Figure 2: Steady-state characteristics. ( a ) Output characteristics for V G varying from 0 (top curve) to +0.5 V (bottom curve) with a step of +0.1 V. ( b ) Transfer curve for V D =−0.6 V, and the associated transconductance. Full size image The transconductance is shown in Fig. 2 to stay above 1 mS over the entire range of applied gate voltage and to reach a peak value of g m =2.7 mS at V G =0.275 V. Devices of similar channel dimensions show a peak g m =2.2±0.8 mS ( N =12). The OECT of Fig. 2 is therefore typical and all subsequent data presented here are for this device, unless otherwise mentioned. The best performing device ( L =10 μm, W =10 μm) shows a transconductance of 4.0 mS ( Supplementary Fig. S1 ). Table 1 contains a comparison of different transistor technologies [15] , [17] , [18] , [19] , [20] , [21] , [22] , [23] , [24] , [25] , [26] , [27] , [28] , [29] , [30] , [31] , [32] , [33] , [34] , [35] , [36] , [37] , [38] , [39] , [40] based on their transconductance. The best PEDOT:PSS-based OECT outperforms all electrolyte- and ionic liquid-gated transistors: it outpaces the highest performing electrolyte-gated graphene transistor by one order of magnitude and silicon transistor by two orders of magnitude. It also performs favourably compared with most solid-state technologies, including, amongst others, oxide-gated graphene [27] , [28] and ZnO [25] . It is only surpassed by III–V semiconductor bulk devices, which, for large channel widths, can yield transconductance values of 30–50 mS [33] , [34] . These devices, which require complex multi-layer fabrication, address a different end of the application’s spectrum. Transconductance is often normalized, depending on the device application or materials family. Normalized to the channel width, the OECT reaches 402 S m −1 , a value only eclipsed by solid-state III–V semiconductor devices, [30] , [31] , [32] , [33] , [34] and is on the same order of magnitude as oxide-gated graphene transistors [27] , [28] . Finally, when the applied voltage is of importance, normalization with respect to V D is used for comparison. The OECT (6,700 μS V −1 ) again compares favourably with all other devices. Table 1 Comparison of the transconductance of various transistors. Full size table Frequency dependence of the transconductance The frequency response of the device shown in Fig. 2 was obtained by measuring the small-signal transconductance. A 100 mV peak-to-peak oscillation was superimposed on the gate bias, and the transconductance was determined by the amplitude ratio between the drain current oscillations and the corresponding input sine wave. 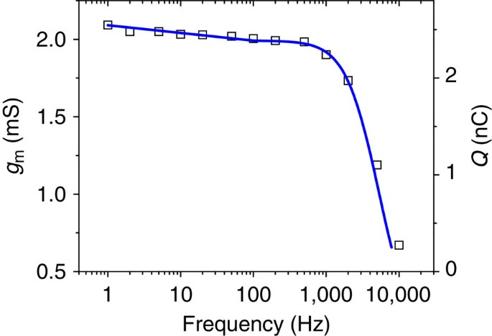Figure 3: Frequency dependence of the transconductance. The device was biased withVD=−0.6 V andVG=0.3 V, and an additional 100 mV peak-to-peak gate voltage oscillation was applied to measure the small-signal transconductance (open squares). The solid line shows the ionic charge injected in the channel. Figure 3 shows that the small-signal transconductance stays close to the DC value up to a frequency of ~1 kHz. This is consistent with the temporal response of the drain current upon the application of a voltage pulse at the gate, which is of the order of 100 μs ( Supplementary Fig. S2 ). This behaviour can be understood by considering the fact that OECTs consist of two circuits [16] : the ionic one, in which ions are transported between the electrolyte and the channel, and the electronic one, in which holes are transported in the PEDOT:PSS channel between the source and the drain. Accordingly, the response time of an OECT can be limited either by ion transport in the ionic circuit, or by the transit time of holes in the PEDOT:PSS channel. The latter was estimated by driving the OECT with constant gate current, I G , and measuring its response time, which, in this case, is solely dependent on the hole transit time, τ e (ref. 16 ): Figure 3: Frequency dependence of the transconductance. The device was biased with V D =−0.6 V and V G =0.3 V, and an additional 100 mV peak-to-peak gate voltage oscillation was applied to measure the small-signal transconductance (open squares). The solid line shows the ionic charge injected in the channel. Full size image This relationship was found to hold in the OECTs presented here ( Supplementary Fig. S3 ), yielding τ e =12.6 μs, a value that indicates that hole transport in the channel is not the limiting factor. This is also consistent with the fact that the response time of the OECTs was found to be dependent on the type of ion in the electrolyte ( Supplementary Fig. S4 ). It should be noted that the hole drift mobility that corresponds to this transit time is 0.05 cm 2 V −1 s −1 . The temporal response of the ionic circuit was evaluated by measuring the impedance, Z , of the channel/electrolyte interface ( Supplementary Fig. S5 ) and calculating the ionic charge, Q , injected in the channel. The latter was derived as: where I G =V G /|Z| , and V G was taken to be the same sinusoidal excitation used to measure the small-signal transconductance (100 mV peak-to-peak). The injected ionic charge is shown in Fig. 3 as a solid line. It shows the same behaviour as the transconductance, signifying that the frequency response of the OECT is dominated by the process of ion transport between the electrolyte and the channel. The agreement between g m and Q is not accidental: Bernards et al . [16] showed that the drain current in an OECT is proportional to the ionic charge injected in the channel. A modulation of the gate voltage will lead to a modulation of this charge, and hence, g m will be proportional to Q . Resistance to mechanical deformation In addition to showing a high transconductance, OECTs display a broad range of practically desirable traits that many of the other technologies cannot achieve, such as ease of fabrication, compatibility with mechanically flexible substrates and resistance to aggressive mechanical deformation. 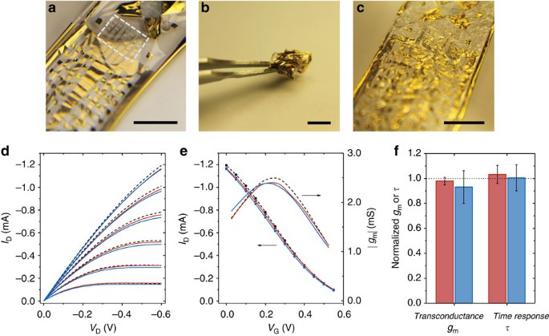Figure 4: Resistance to mechanical deformation. (a) An array of devices removed from the sacrificial glass substrate (active area shown as boxed region). (b) The array aggressively crumpled. (c) The array un-crumpled back to a flat sheet. Scale bar, 1 cm. (d) Output characteristics and (e) transfer characteristics for the same device as-prepared (black), after peeling (red) and after crumpling (blue). (f) Transconductance and time response for devices after peeling (red), and after crumpling (blue), normalized to the performance of each device as-prepared (Error bars represent standard deviation of normalized values forN=16 devices, on three different substrates). Figure 4 shows an array of devices that was peeled-off from its glass sacrificial substrate, crumpled, and then un-crumpled back to a flat sheet. The peeled-off devices had a thickness of ~4 μm, with the PEDOT:PSS channel and the Au interconnects in the neutral mechanical plane. Characterization before and after crumpling showed that the devices could withstand the trial without a significant change in performance. Figure 4d shows the electrical characteristics of one of the devices in this array ( L =10 μm, W =10 μm) as-prepared (black), after peel-off from its glass sacrificial substrate (red), and after crumpling (blue), revealing that the transconductance remains practically unchanged. Over 16 devices tested on three different substrates showed little variation in transconductance and time response when exposed to such a harsh handling ( Fig. 4f ). Figure 4: Resistance to mechanical deformation. ( a ) An array of devices removed from the sacrificial glass substrate (active area shown as boxed region). ( b ) The array aggressively crumpled. ( c ) The array un-crumpled back to a flat sheet. Scale bar, 1 cm. ( d ) Output characteristics and ( e ) transfer characteristics for the same device as-prepared (black), after peeling (red) and after crumpling (blue). ( f ) Transconductance and time response for devices after peeling (red), and after crumpling (blue), normalized to the performance of each device as-prepared (Error bars represent standard deviation of normalized values for N =16 devices, on three different substrates). Full size image The absence of a dielectric between channel and electrolyte in OECTs allows ions to be injected into the former and gives rise to a response that is determined by the volume of the channel. This is in contrast to electrolyte-gated field-effect transistors, where accumulation of charge at the interface between electrolyte and gate insulator (or semiconducting channel) determines the response. This fact is reflected in the magnitude of the charge injected in the channel, which, at low frequencies, is equal to ~2.5 nC ( Fig. 3 ). This corresponds to 7.8 × 10 20 ions. cm −3 , a value within the range of the doping level of PEDOT:PSS (ref. 41 ), indicating that the transistor operates close to limit of complete dedoping. As expected, the transistor performance can be tuned by adjusting the channel volume. Making the channel thinner, for example, can lead to faster response, as dedoping it requires a smaller number of ions. At the same time, the drain current (hence its modulation upon gating) decreases, leading to a lower transconductance. Indeed, a device with a PEDOT:PSS channel ( L =5 μm, W =10 μm) that was 100 nm thick had a response time of 37 μs and a transconductance of 1.6 mS ( Supplementary Fig. S6 ). In addition to adjusting channel volume, OECT performance can potentially be further improved through the synthesis of new materials. Conducting polymers with a higher capacity to store charge, for example, would lead to devices with a higher transconductance. The design of such polymers is also the focus of contemporary research on batteries [42] , a synergy that has the chance to lead to the development of new high-performance materials for electrochemical devices. In terms of response time, little is known about ion transport in conducting polymers. Recent measurements by Stavrinidou et al . [43] showed that ion mobility in PEDOT:PSS depends on water uptake: pristine PEDOT:PSS films in contact with aqueous electrolytes were found to swell and support transport of small ions with the same mobility as in water. Cross-linking the films diminished their ability to uptake water and decreased ion mobilities. As the relationships between conducting polymer structure and ion transport properties become more established in the future, synthesis of new materials might yield OECTs that operate at higher frequencies. Finally, beyond geometry and materials, the application of a higher drain voltage increases transconductance, but there is a limit of ~1 V to the voltage that can be applied in an aqueous electrolyte before electrolysis takes place. Some ionic liquids and gels enable higher voltage operation, hence higher performance [12] . The OECT, when biased as shown in Fig. 1 , acts as a transconductance amplifier that converts a voltage modulation at the gate to a modulation of the drain current. Considering a biasing point of V D =−0.6 V and V G =0.275 V for the device of Fig. 2 , an increase of the input (gate) voltage of 100 mV will result in a change of 270 μA in the output (drain) current. At the same time, the input current remains below 10 nA, increasing by only 2 nA. Therefore, the input signal power is 100 mV × 2 nA=200 pW and the output signal power is 0.6 V × 270 μA=162 μW, yielding a power amplification of 59 dB. Such high power amplification can be harnessed in biosensing applications, which require operation in an aqueous electrolyte and are operated in a DC mode. Interfacing with electrically active cells and tissues is another potential application for OECTs. Extracellular signals, which are of order of 100 μV, can be easily discernible by the OECT, whose transconductance at the frequency of action potentials (1 kHz) is still sufficiently large to ensure significant power amplification. In all these applications, a significant advantage of OECTs as a first stage amplifier is that the input signal is transduced and amplified right at the interface and is hence not corrupted by noise from external wiring and circuitry. In fact, we recently showed that OECTs can record brain activity in vivo with a higher signal-to-noise ratio than electrodes [44] . Moreover, the fact that OECTs work even after being mechanically deformed opens up a new world of opportunities for devices ranging from smart bandages to intelligent clothing. Device fabrication The fabrication process, similar to that reported previously [45] , included the deposition and patterning of parylene, metal and PEDOT:PSS. A parylene-C film was deposited on a glass slide using a SCS Labcoater 2 to a thickness of 2 μm (at which the layer is pinhole-free). This layer of parylene was fixed on the glass slide using 3-(trimethoxysilyl)propyl methacrylate as an adhesion promoter. Avoiding the adhesion promoter allowed the devices to be peeled-off after fabrication. An additional 2 μm thick layer of parylene was used to insulate the metal pads from the electrolyte. It was patterned with AZ9260 photoresist and reactive ion etching by an O 2 plasma using an Oxford 80 plus. Metal pads and interconnects were patterned by a lift-off process, using S1813 photoresist, exposed to UV light using a SUSS MBJ4 contact aligner, and developed using MF-26 developer. Five nanometre of titanium and 100 nm of gold were then deposited using a metal evaporator, and metal lift-off was performed using acetone. For the preparation of the PEDOT:PSS films, 20 ml of aqueous dispersion (PH-1000 from Heraeus Clevios GmbH), 1 ml of ethylene glycol, 50 μl of dodecyl benzene sulphonic acid were mixed and sonicated before spin-coating. The films were subsequently baked at 140 °C for 1 h and were immersed in deionized water to remove any excess low molecular weight compounds. Electrical characterization All characterization was done using a solution of 100 mM NaCl in DI water as the electrolyte and a Ag/AgCl wire (Warner Instruments) as the gate electrode. The electrical characteristics of the OECTs were measured with two VA10 transimpedance amplifiers (NPI) and customized LabVIEW software. Impedance measurements were carried out using an Autolab PGSTAT 128N. The OECT channel was used as the working electrode (source and drain connected together), while a bridge electrode was used as the reference and a Pt foil was used as the counter electrode. The electrolyte was the same as for the OECT characterization. A modulation with amplitude of 10 mV was applied, while the bias was varied between 0.4 V and −0.4 V, and found to make no difference in the recorded impedance. How to cite this article: Khodagholy, D. et al . High transconductance organic electrochemical transistors. Nat. Commun. 4:2133 doi: 10.1038/ncomms3133 (2013).